Fast electrical switching of orbital angular momentum modes using ultra-compact integrated vortex emitters The ability to rapidly switch between orbital angular momentum modes of light has important implications for future classical and quantum systems. In general, orbital angular momentum beams are generated using free-space bulk optical components where the fastest reconfiguration of such systems is around a millisecond using spatial light modulators. In this work, an extremely compact optical vortex emitter is demonstrated with the ability to actively tune between different orbital angular momentum modes. The emitter is tuned using a single electrically contacted thermo-optical control, maintaining device simplicity and micron scale footprint. On–off keying and orbital angular momentum mode switching are achieved at rates of 10 μs and 20 μs respectively. The orbital angular momentum (OAM) of light represents an additional degree of freedom for light beams and single photons over those used in conventional optical systems (such as, polarization and wavelength) [1] , [2] . OAM is defined in an unbounded infinite-dimensional space, therefore it is possible to encode a much larger amount of information in this degree of freedom, offering orders of magnitude greater transmission capacity [3] , [4] , [5] , [6] , as well as allowing for higher-security communication protocols [7] , [8] , [9] , [10] . This makes OAM very attractive for applications in future optical communication and quantum key distribution (QKD) systems. To fully access the benefits of the OAM degree of freedom, devices that can rapidly switch between OAM modes are highly desirable. For classical communication systems, multiplexing and demultiplexing of OAM modes has recently led to record-breaking data communication rates both in free space [3] and in optical fibres [4] . In a similar manner to the evolution of wavelength division-multiplexed systems, the future advancement of OAM-based telecommunication systems will require OAM routing flexibility and reconfigurability with components that can perform the fast switching of OAM data channels [5] , [11] . For quantum communication systems, current QKD schemes, relying on polarization encoding, suffer a tight bound on the error tolerance due to the limits on the amount of information that can be sent per photon [8] , [9] . OAM-based QKD systems show the promise of providing an enhanced tolerance to errors, and therefore the potential for a quantum communication channel that is more robust against eavesdropping [7] , [8] , [9] , [10] . The development of fast OAM switching devices is of great importance for OAM-based QKD systems, because the key generation rate of the systems is currently limited by the switching speed of OAM states in such devices. The commonly used OAM switching or manipulation tools, including spatial light modulators (SLMs) [12] , [13] and q-plates [14] , [15] are slow to respond with the best switching rates of the order of 1 kHz. Higher switching rates have been reported by using digital micro-mirror devices [16] , combining q-plates with electro-optical modulators, or combining SLMs with acousto-optic modulators [17] . However, all of these approaches rely on large scale optical components with limitations in terms of cost, stability and scalability. Recently, several integrated photonic circuits have been demonstrated for the generation and measurement of OAM carrying beams [18] , [19] , [20] . These circuits rely on complicated phase-sensitive arrayed waveguide structures with a large number of electrical contacts for phase calibration. Here, based on our previous work [21] , we report an ultra-compact tunable integrated OAM device on silicon-on-insulator material, capable of actively on–off keying OAM modes at record rates of 10 μs and switching OAM modes at record rates of 20 μs. A single electrically contacted thermo-optical control is used to achieve rapid switching of OAM modes. In addition, the emitted OAM modes show high mode purities within the range of 86–99%. This work paves the way for a scalable integrated silicon photonic platform for high-speed switching of the OAM modes of light on-chip. Principle We have previously presented an integrated device for the emission of optical beams with well-defined OAM modes [21] . The operation principle of the device is based on the coupling of whispering gallery modes (WGM) of a microresonator to free-space propagating OAM modes through the use of an angular grating embedded within the microresonator. The generated OAM mode order, l , is defined by the resonant WGM order, p , and the number of scattering elements in the ring, q , as: This device benefits from extremely simple operation and compact size, requiring only a ring resonator and a bus waveguide for coupling of the input optical signal. Different OAM modes can then be addressed by aligning the input wavelength to different resonances of the device. In this paper, a complimentary method by which the emitted OAM modes at a fixed wavelength can be actively modulated is presented, using only a single electrical component. The resonant WGM wavelengths, λ R , of a ring resonator can be defined as: where n e is the wavelength-dependent effective index of the waveguide and L c is the geometrical roundtrip length of the ring. Therefore, in a resonator with q scattering elements, the emitted OAM mode order l = p − q will vary for each λ R as: By exercising control over the waveguide effective index, on-chip modulation of the generated OAM modes, at a fixed wavelength, can be achieved. Tuning of silicon devices through refractive index modulation has been implemented using thermal [22] or carrier-induced effects [23] . In this work, a resistive heater device was designed to create a thermal change of refractive index in the waveguide core, and hence tune the WGM mode and emitted OAM mode. 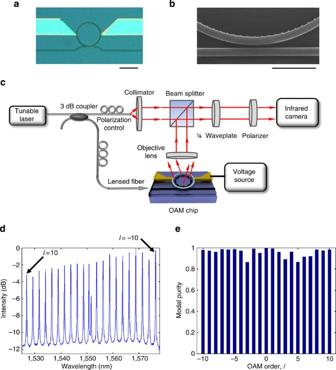Figure 1: Tunable integrated orbital angular momentum devices. (a) Optical and (b) scanning electron microscopy (SEM) images of the fabricated device. The SEM image was taken before fabrication of the electrical components. Scale bars, 50μm and 2μm foraandbrespectively. (c) The experimental setup for investigating the phase structure of the radiated beam from the device. (d) Excitation spectrum of the vortex beam emitter (froml=−10 tol=10). (e) Mode purities measured as a function of orbital angular momentum orderl-value. Figure 1a,b shows a micrograph and a scanning electron microscopy image of the tunable vortex beam emitter. The metal resistive line was defined concentrically with the ring resonator, with a slightly larger radius than the silicon ring. This radial offset, while still allowing significant thermo-optic tuning, ensured that the emitted beam did not overlap the absorbing metallic structure. As the resistive heater width is <1 μm in dimension, the compact footprint of the device is retained, and furthermore, the use of a single electrical connection for device control maintains the essential simplicity of the emitter, allowing for the multiplexing of many individually controlled emitters in an array. Figure 1: Tunable integrated orbital angular momentum devices. ( a ) Optical and ( b ) scanning electron microscopy (SEM) images of the fabricated device. The SEM image was taken before fabrication of the electrical components. Scale bars, 50μm and 2μm for a and b respectively. ( c ) The experimental setup for investigating the phase structure of the radiated beam from the device. ( d ) Excitation spectrum of the vortex beam emitter (from l =−10 to l =10). ( e ) Mode purities measured as a function of orbital angular momentum order l -value. Full size image Emission spectrum and mode purity The measurement setup used to assess the emitted OAM beam mode order is shown in Fig. 1c . Simple emission spectra were measured by scanning the tunable laser wavelength and monitoring the full measured power at the infrared (IR)-camera position using a photodetector while the reference beam was blocked. The OAM beam was coupled through the polarization filter, consisting of a quarter-wave plate and a polarizer, before interference with a co-propagating Gaussian reference beam on the camera. The left hand circularly polarized (LHCP) or right hand circularly polarized (RHCP) component of the beam was converted to a linear polarized beam with OAM value of l −1 or l +1, depending on the relative angle between the axis of the quarter-wave plate and the polarizer. Therefore, spiral interferograms, with number of arms equal to either l −1 or l +1, were obtained. Figure 1d shows the emitted excitation spectrum of the device obtained by scanning the wavelength of the input laser, while the heater is un-biased. As previously shown [21] , the mode splitting close to 1,550 nm is the signature of the l =0 mode, with positive and negative values of l extending to shorter and longer wavelengths respectively. The emission efficiencies at various resonances were measured to be between 6.7 and 14.9%. The device is designed in such a way that the forward travelling wave is coupled to the l th OAM mode (see supplementary materials in ref. 21 ). However, the strong backscattering of the silicon waveguide and the grating itself inside the microresonator couple the forward and backward travelling waves [24] , [25] , and the backscattered wave subsequently couples to the − l vertically emitted beam. Therefore, in addition to the expected value of the OAM beam, l, at each resonant wavelength, the opposite OAM value, − l , is also observed experimentally. The measured mode purities of 21 OAM modes are shown in Fig. 1e , which are defined by Power l /(Power l +Power −l ) [13] , where Power l and Power −l are the power of the OAM beams with a value of l and −l respectively (see further details in the Methods). Following the methods in ref. 13 , the mode purities across the spectrum were measured to range from 86 to 99%. Static characterization To tune the device, a voltage was applied across the heater terminals. 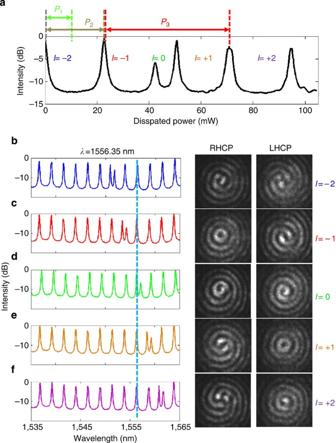Figure 2: Static characterization of the tunable integrated orbital angular momentum device. (a) Measured emission from the device withλ=1556.35 nm and variable dissipated power on the resistive heating element. (b–f) Measured excitation spectra of the device with various heater voltages and the measured interferograms (forλ=1,556.35 nm) of the two polarization components of the beam with a Gaussian reference beam. Figure 2a shows the relationship between the vertical emission intensity from the device and the power dissipated in the resistive heater when the injected light wavelength is kept constant at 1,556.35 nm. From a starting position on resonance at l =−2, the resonator was firstly tuned off resonance so that the emission was cut, then subsequent OAM modes were tuned across the injected light wavelength with a linear relationship between dissipated power and OAM mode order. The reconstructed spectrum illustrates that within this range, with a given fixed input wavelength, the device can be tuned across 5 OAM modes, with the relative emission efficiency varying by <2 dB. Figure 2b–f shows the measured excitation spectra (while the injected signal wavelength was scanned) as a function of dissipated power in the resistive heater. In addition, interferograms are presented that were obtained by beating the emitted OAM beam with a Gaussian reference beam on an IR camera at a wavelength of 1,556.35 nm. Figure 2: Static characterization of the tunable integrated orbital angular momentum device. ( a ) Measured emission from the device with λ =1556.35 nm and variable dissipated power on the resistive heating element. ( b – f ) Measured excitation spectra of the device with various heater voltages and the measured interferograms (for λ =1,556.35 nm) of the two polarization components of the beam with a Gaussian reference beam. Full size image Dynamic characterization To demonstrate dynamic control over the OAM values of the emitted beam, 10 kHz square-wave driving signals ( Fig. 3a ), with different peak dissipation power values ( P 1 , P 2 and P 3 in Fig. 2a ), were applied to the device. For example, in the case of P 1 , a 10 mW peak power square wave was applied to the device to shift the ring out of resonance, and so, effectively, turn off the vortex beam emission. The measured trace in Fig. 3b shows on–off keying of the emission signal corresponding to the driving signal, with a measured rise-time of 10 μs and a fall-time of 1.4 μs. 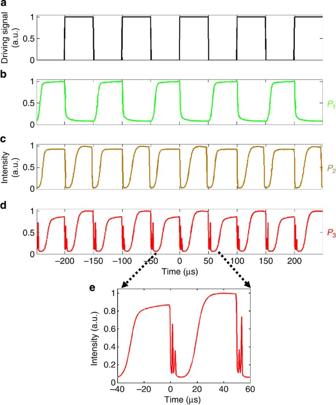Figure 3: Dynamic characterization of the tunable integrated orbital angular momentum devices. (a) Normalized input electrical driving signal. Measured optical signal for (b) on–off keying, (c) switching betweenl=−2 andl=−1 (d) and (e) switching betweenl=−1 andl=+1. Figure 3: Dynamic characterization of the tunable integrated orbital angular momentum devices. ( a ) Normalized input electrical driving signal. Measured optical signal for ( b ) on–off keying, ( c ) switching between l =−2 and l =−1 ( d ) and ( e ) switching between l =−1 and l =+1. Full size image In addition to on–off keying of the vortex emission, real-time switching between the OAM modes can also be achieved. In this case the high and low values of the driving signal can be set to correspond to different OAM modes. Figure 3c,d shows the cases for driving signals of 0–23 mW and 23–70 mW, corresponding to OAM mode switching between l =−2 and l =−1 and l =−1 and l =+1, respectively, given as P 2 and P 3 in Fig. 2a . For the measurement of Fig. 3d where the signal sweeps across the double peaked l =0 modes, brief spikes in the temporal response corresponding to those resonances are clearly visible and are shown in greater detail in Fig. 3e , where the asymmetry of the l =0 mode amplitudes can be used to identify the direction of the spectral mode tuning with time. In this case the switching time was measured as 20 μs. Finally, to unambiguously demonstrate the real-time switching between different OAM modes, the experimental setup illustrated in Fig. 4a was constructed. In this arrangement, the driving signal to the vortex beam emitter was also connected to a two port optical switch. With output port 1 of the optical switch aligned with the input waveguide of the integrated chip, the electrical signal synchronized an on–off keying of the optical switch with the OAM switching of the device. Therefore, as for the continuous wave injection case, an interferogram of the emitted vortex beam can be measured corresponding to one state of the switching. The second state can then be measured by simply aligning port 2 of the optical switch with the input waveguide of the chip. Both of these interferograms are shown in Fig. 4b,c , along with measured optical signals from the setup. In this case the electrical signal is 0–23 mW corresponding to an OAM mode switching between l =−2 and l =−1. The measured interferograms, created through interference between the linearly polarized beams converted from RHCP and Gaussian reference beams, clearly show the expected spiral patterns associated with the predicted OAM states. 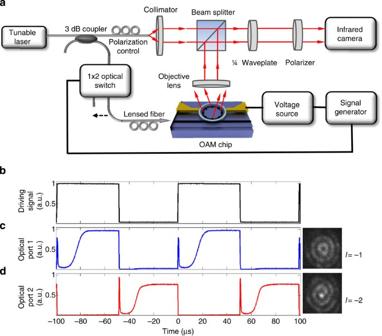Figure 4: Real-time switching measurement. (a) Schematic of the measurement setup for capturing interferograms of the orbital angular momentum mode switching. (b) Normalized electrical driving signal for switching betweenl=−2 andl=−1. (c,d) optical signals measured in the time domain with the optical switch coupled to port 1 or port 2 respectively, along with the measured interferograms. Figure 4: Real-time switching measurement. ( a ) Schematic of the measurement setup for capturing interferograms of the orbital angular momentum mode switching. ( b ) Normalized electrical driving signal for switching between l =−2 and l =−1. ( c , d ) optical signals measured in the time domain with the optical switch coupled to port 1 or port 2 respectively, along with the measured interferograms. Full size image We report on an ultra-compact silicon integrated device capable of rapidly tuning the OAM modes of emitted light. This is the first demonstration of fast OAM states switching on-chip, and the switching rate of the device is one to two orders of magnitude faster than previously demonstrated with bulk-optics approaches. These switching rates provide an integrated device that can be used in applications including optical data burst and packet switching [26] and quantum encryption [8] . Even faster switching among OAM modes, in the order of 100 ns, can be achieved by further optimizing heater designs [27] and nano-to-picosecond switching times are possible by using carrier injection [23] . Compared with other photonic integrated circuits with complicated phase-sensitive arrayed waveguide structures, the tuning of the OAM modes is achieved by the integrated micro-sized heater, which maintains device simplicity and micron scale footprint. Following the methods of Gibson et al. [13] , the mode purities of the generated OAM modes were measured to range from 86 to 99% at various resonances of the devices, with the undesired OAM mode contribution arising from the backward travelling wave inside the device due to backscattering in the silicon waveguide [24] , [25] . In summary, the fully on-chip and single contact control of the OAM device opens up a wide range of possibilities for applications in sensing and manipulation [28] , [29] , [30] , telecommunications [3] , [4] , [5] , [6] and quantum optics [8] , [9] , [10] , [31] , [32] , [33] , [34] . Devices fabrication and characterization The micro-ring optical vortex emitter was fabricated on a silicon-on-insulator wafer with 220-nm-thick silicon core and 2 μm buried oxide layer. The ring was defined with a radius of 36.6 μm and q =360 grating elements with a square perturbation cross-section of 60 nm side length. The device was patterned using direct write electron beam lithography into a Hydrogen Silsequioxane resist layer. On development, the resist pattern was used as a hard mask for Reactive Ion Etching of the silicon layer. The silicon device was subsequently coated with a 900-nm-thick layer of SiO 2 as a buffer layer between the device and the metal contact layers. The resistive heater was formed using a lift-off technique with 50 nm of NiCr. The electrical transmission lines to the heater element was similarly patterned with a 200-nm-thick Au layer. Finally, wire bonding was carried out for electrical contacting the on-chip transmission lines. The resistive heater had a series resistance of 1.5 kΩ and was driven using a constant voltage power supply and an Agilent 33120A function generator. For all emission measurements, light from a tunable laser (Photonetics, Tunics-BT) was coupled via a lensed optical fibre to the input waveguide of the silicon chip. The vertical emission of the ring device was collected with a microscope objective and imaged onto an NIR camera (Hamamatsu Photonics). For the interferogram measurements, a portion of the source laser light was coupled into a free space Gaussian beam, which was subsequently coaligned with the beam from the vortex emitter for interference on the camera. Emitted OAM beams were coupled to an InGaAs-amplified photodetector for the dynamic characterization. Mode purity measurement An experimental setup based on a SLM (HOLOEYE, PLUTO 1,550 SLM), as shown in Fig. 5 , was used to study the mode purity of the emitted OAM beam from the device. After going through the polarization filter, the RHCP or LHCP component of the beam was converted to a linearly polarized beam with OAM value of l −1 or l +1, depending on the relative angle between the axis of the quarter-wave plate and the polarizer. The polarization filter was used as the SLM can only operate on linearly polarized light. The OAM order of the linearly polarized beam was then analyzed by changing the order of the holographic pattern on the SLM (number of phase dislocations on the Y-branch hologram). If the order of the SLM hologram, H , is the negative of the OAM value of the beam then the resulting beam has planar phase fronts and therefore can be focused into a bright spot at the centre of the image. The on-axis intensity of each beam was determined from the images on an IR CCD array [13] . As an example, the on-axis intensities distribution of the LHCP component of the OAM beams with the expected OAM order of l =−10 is shown in Fig. 6 . The two dominant peaks are the on-axis intensities where the order of the holographic patterns are H =11 and H =−9 respectively, and coincide with the desired OAM order, l =−10, and the OAM order from backscattering mode, l =10. The mode purity of the OAM beam with l =−10 is measured at 97%. Figure 6 also shows intensity profiles of the beams after the SLM recorded by the IR camera and the corresponding holographic phase structures on the SLM. 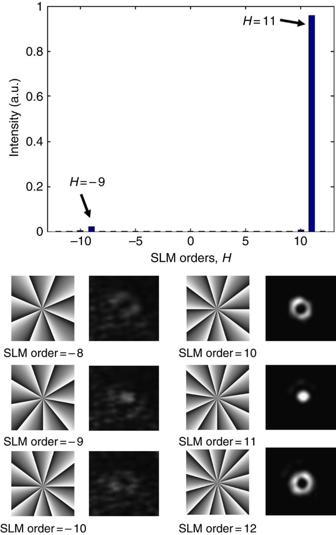Figure 6: Mode purity measurement. On-axis intensities distribution of the left hand circularly polarized component of the orbital angular momentum beams withl=−10. Intensity profiles after the spatial light modulator (SLM) and the corresponding holographic phase structures on the SLM. 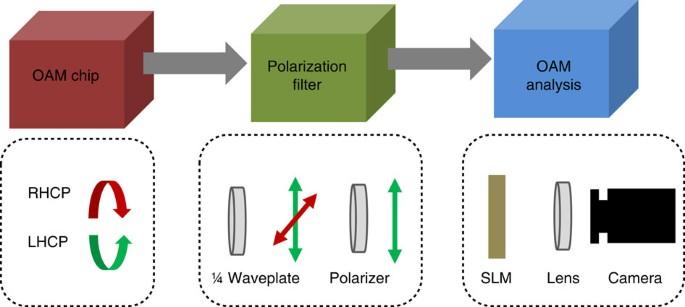Note that the mode purity of the beam with l =0 is 100%, due to the indistinguishablity between the forward and backward-coupled beams at l =0. Figure 5: Schematic diagram of the orbital angular momentum mode purity measurement. Right and left hand circularly polarized components of the on-chip generated optical vortex beam are converted to horizontal and vertical linearly polarized beams. The selected linearly polarized beam is coupled through a spatial light modulator onto an IR CCD camera to capture the intensity distribution of the modulated beam. By varying the order of the spatial light modulator holographic pattern the power in each orbital angular momentum mode can be measured as a function of the on-axis intensity. Figure 5: Schematic diagram of the orbital angular momentum mode purity measurement. Right and left hand circularly polarized components of the on-chip generated optical vortex beam are converted to horizontal and vertical linearly polarized beams. The selected linearly polarized beam is coupled through a spatial light modulator onto an IR CCD camera to capture the intensity distribution of the modulated beam. By varying the order of the spatial light modulator holographic pattern the power in each orbital angular momentum mode can be measured as a function of the on-axis intensity. Full size image Figure 6: Mode purity measurement. On-axis intensities distribution of the left hand circularly polarized component of the orbital angular momentum beams with l =−10. Intensity profiles after the spatial light modulator (SLM) and the corresponding holographic phase structures on the SLM. Full size image How to cite this article: Strain, M. J. et al. Fast electrical switching of orbital angular momentum modes using ultra-compact integrated vortex emitters. Nat. Commun. 5:4856 doi: 10.1038/ncomms5856 (2014).